Metal-free dehydropolymerisation of phosphine-boranes using cyclic (alkyl)(amino)carbenes as hydrogen acceptors The divalent carbene carbon centre in cyclic (alkyl)(amino)carbenes (CAACs) is known to exhibit transition-metal-like insertion into E–H σ-bonds (E = H, N, Si, B, P, C, O) with formation of new, strong C–E and C–H bonds. Although subsequent transformations of the products represent an attractive strategy for metal-free synthesis, few examples have been reported. Herein we describe the dehydrogenation of phosphine-boranes, RR’PH·BH 3 , using a CAAC, which behaves as a stoichiometric hydrogen acceptor to release monomeric phosphinoboranes, [RR’PBH 2 ], under mild conditions. The latter species are transient intermediates that either polymerise to the corresponding polyphosphinoboranes, [RR’PBH 2 ] n (R = Ph; R’ = H, Ph or Et), or are trapped in the form of CAAC-phosphinoborane adducts, CAAC·H 2 BPRR’ (R = R’ = t Bu; R = R’ = Mes). In contrast to previously established methods such as transition metal-catalysed dehydrocoupling, which only yield P-monosubstituted polymers, [RHPBH 2 ] n , the CAAC-mediated route also provides access to P-disubstituted polymers, [RR’PBH 2 ] n (R = Ph; R’ = Ph or Et). Polymers that feature p -block elements other than carbon in the main chain are interesting materials due to their potential uses as elastomers, etch resists in lithography, polyelectrolytes, ceramic precursors and in optoelectronics [1] , [2] , [3] , [4] . Earlier syntheses of inorganic polymers were achieved by the use of polycondensation and ring-opening methods [1] , [2] , [5] . Access to stable yet reactive, polymerisable, multiply bonded p -block monomers required for addition polymerisation remains a major challenge in the synthesis of inorganic polymers [6] , [7] , [8] . More recently, metal-catalysed coupling routes have been developed for accessing a broad range of inorganic macromolecules and materials [2] , [9] , [10] , [11] , [12] , [13] , [14] . In this context catalytic dehydrocoupling between main-group substrates has been shown to be a versatile method for the general formation of E–E′ bonds, which can be also used to access polymers via catalytic dehydropolymerisation [15] , [16] , [17] , [18] , [19] , [20] . Polyphosphinoboranes attracted initial interest in the 1950s as a result of their potential as flame-retardant materials with high thermal stability [21] , [22] , [23] . However, attempts to dehydrocouple phosphine-borane adducts under thermal conditions yielded either low molecular weight or poorly soluble materials, which lacked convincing structural characterisation by modern standards [2] , [24] , [25] . Since 1999 a rhodium-catalysed dehydrocoupling approach to prepare soluble, high-molecular-weight (P-monosubstituted)polyphosphinoboranes has been available [26] , [27] , [28] . Examples of iron and iridium-catalysed dehydrocouplings have also been reported as routes to high-molecular-weight poly(arylphosphinoboranes) (Fig. 1a ) [29] , [30] . Notably, these transition metal-catalysed protocols all require forcing conditions (≥100 °C, ≥20 h) and their scope is currently limited to the dehydrocoupling of primary arylphosphine-boranes, RPH 2 ·BH 3 (R = aryl). More recently, from our collaboration with Scheer and co-workers [31] , [32] , a metal-free synthesis of polyphosphinoboranes through the thermolysis of amine-stabilised phosphinoboranes, RR′PBH 2 ·NMe 3 , was reported to proceed under milder conditions 22–40 °C. This route successfully produced high-molecular-weight poly- tert -butylphosphinoborane, [ t BuHPBH 2 ] n , presumably via the monomeric phosphinoborane [ t BuHPBH 2 ]. However, the precursors are challenging to prepare and attempts to access the P-disubstituted poly(diphenylphosphinoborane), [Ph 2 PBH 2 ] n , by the thermolysis of Ph 2 PBH 2 ·NMe 3 , yielded only very-low-molecular-weight oligomers [Ph 2 PBH 2 ] x ( x ≤ 6) (Fig. 1b ). The development of convenient and efficient dehydrocoupling of secondary phosphine-borane adducts to give the corresponding polymers therefore remains an open challenge. Herein, we demonstrate the successful use of the carbene centres of cyclic (alkyl)(amino)carbenes (CAACs) to mediate this process. Fig. 1 Synthesis of polyphosphinoboranes. a , b Current methods of synthesis and c proposed CAAC-mediated dehydrogenation Full size image CAACs are analogues of N -heterocyclic carbenes (NHCs) with one of the electronegative amino substituents replaced by a strong σ-donating alkyl group, which simultaneously increases the nucleophilicity and electrophilicity at the divalent carbene carbon centre [33] , [34] , [35] , [36] . The resulting small HOMO–LUMO gap of CAACs has allowed E–H (E = H, N, Si, B, P, C, O) bond activation by formal oxidative addition to the carbene carbon centre for a variety of small molecules under mild conditions, with this process giving products featuring a H–C(sp 3 )–E moiety [37] , [38] , [39] , [40] , [41] , [42] . However, the strength of the resulting C(sp 3 )–H and C(sp 3 )–E σ−bonds disfavours further reactivity of the H–C(sp 3 )–E products, limiting the ability of CAACs to mimic transition metal centres in synthetic utility. We envisioned that a CAAC-mediated dehydrogenation of primary and secondary phosphine-boranes, species that contain both protic P–H and hydridic B–H bonds, may be possible (Fig. 1c ). Dehydrogenation of phosphine-boranes using this strategy leads to reactive phosphinoborane monomers, which, given appropriate substituents at the phosphorus and boron centres, gives soluble oligomeric and polymeric material. Reactivity of carbenes with phosphine-boranes The synthesis of monomeric aminoborane-NHC adducts (NHC-BH 2 NHR) has been reported both through the use of an NHC for ambient temperature dehydrogenation of amine-boranes (RNH 2 ·BH 3 ; R = H, Me) [43] and NHC-induced depolymerisation of poly( N -methylaminoborane) [44] . More recently, analogous species featuring the use of NHCs to stabilise phosphinoborane monomers have been isolated using NHC-induced thermal depolymerisation of polyphosphinoboranes [45] . Consequently, prior to investigating the reactivity of phosphine-boranes with CAACs, we explored the dehydrogenation potential of NHCs. Upon addition of one equivalent of IDipp to a solution of PhPH 2 ·BH 3 in tetrahydrofuran (THF), a homogeneous solution was formed after 10 min, and analysis of the reaction mixture by 31 P and 11 B nuclear magnetic resonance (NMR) spectroscopy showed complete conversion to a new species (δ P = −84.2ppm (br), δ B = −33.4ppm (dq) in THF) (Supplementary Figs. 2 and 3 ). The similarity of these spectral features to those observed for Li[PhPHBH 3 ] (δ P = −93.8ppm (d), δ B = −34.6ppm (dq) in THF) [46] , an analogous compound with a different cation, is consistent with deprotonation of PhPH 2 ·BH 3 by IDipp to yield the salt [IDippH][PhHPBH 3 ] ( 1a ) (Fig. 2a ). The formation of this salt was further confirmed by an independent synthesis via a metathesis reaction in THF between [IDippH]Cl and Li[PhHPBH 3 ]. This showed 11 B and 31 P NMR spectral features that matched those assigned to 1a along with precipitation of LiCl (Fig. 2b ). The 13 C NMR spectrum of 1a showed no 1 J CP couplings involving the iminium carbon atom, which, together with the downfield chemical shift in the 1 H NMR spectrum of the imidazolium proton (δ H = 10.0ppm) (Supplementary Fig. 1 ), supports an ionic formulation for this species in solution. When Ph 2 PH·BH 3 was reacted with IDipp, the analogous salt [IDippH][Ph 2 PBH 3 ] ( 1b ) was formed (Supplementary Figs. 4 – 6 ) and subsequently characterised using X-ray crystallography (Supplementary Fig. 7 and Supplementary Table 6 ). Fig. 2 Reactivity of IDipp and CAAC Me with phosphine-boranes. a Synthesis of 1a and 1b by deprotonation of the phosphine-borane using IDipp; b synthesis of 1a and 1b using salt metathesis route; c synthesis of 3a through oxidative addition of PhPH 2 ·BH 3 ; d synthesis of 3a through stepwise reaction of PhPH 2 , then BH 3 ·THF; and e synthesis of 3a through salt metathesis route Full size image Next, we attempted the analogous reaction with a CAAC as the smaller HOMO–LUMO separation of CAACs renders them potentially better candidates for E–H bond activations. The P–H activation of PhPH 2 ·BH 3 by one equivalent of CAAC Me (Fig. 2c ) occurred readily at 22 °C in THF to give 3a , which exists as two diastereomers ( 3a′ and 3a″ ). The identity of 3a was initially established based on a distinctive doublet of quartet of doublets coupling pattern observed in the 1 H NMR spectrum for the P–H protons (Supplementary Figs. 8 – 10 ). This assignment was further corroborated by an independent synthesis via a stepwise procedure involving oxidative addition of PhPH 2 to the carbene centre in CAAC Me to yield 2a (as a mixture of diastereomers each with indistinguishable enantiomers by NMR), followed by the addition of BH 3 ·THF to give 3a (Fig. 2d ). The two diastereomers of 3a were also formed immediately upon combining Li[PhHPBH 3 ] and [CAAC Me H]Cl through elimination of LiCl (Fig. 2e ). In contrast to the results obtained in the reaction of [IDippH]Cl and Li[PhPHBH 3 ] above (Fig. 2b ), the lower steric hindrance and greater π-acidity [36] of the cation [CAAC Me H] + leads to the formation of a molecular species with a distinct P–C bond, rather than the corresponding iminium salt [CAAC Me H][PhPHBH 3 ]. The molecular formulation of 3a is supported by the observation of both 1 J CP ( 1 J CP = 41.0 Hz ( 3a′ ), 1 J CP = 38.3 Hz ( 3a″ )) and 2 J HP ( 2 J HP = 4.2 Hz ( 3a′ ), 2 J HP = 5.8 Hz ( 3a″ )) coupling constants in the 13 C and 1 H NMR spectra. Attempts to crystallographically characterise 3a were unsuccessful as solutions in THF (0.10 M) spontaneously decomposed to a mixture of poly(phenylphosphinoborane) [PhHPBH 2 ] n and (CAAC Me )H 2 as shown by 1 H, 11 B and 31 P NMR spectroscopy. Although only sensitive to low molar mass fractions [47] , electrospray ionisation-mass spectrometry (ESI-MS) confirmed the formation of [PhHPBH 2 ] n (up to n = 22) by identifying repeat units of ∆( m/ z) = 122.05 (molecular weight of [PhHPBH 2 ] = 122.05 g mol −1 ). Isolation of pure [PhHPBH 2 ] n was achieved through precipitation of the reaction mixture into cold (−40 °C) hexanes to remove the hydrogenated carbene, (CAAC Me )H 2 (Supplementary Figs. 25 and 26 ), which was also characterised by X-ray crystallography (Supplementary Fig. 27 and Supplementary Table 6 ). In the present case, the eliminated phosphinoborane monomer [PhHPBH 2 ] polymerises, presumably due to the small size of the substituents at P and B. 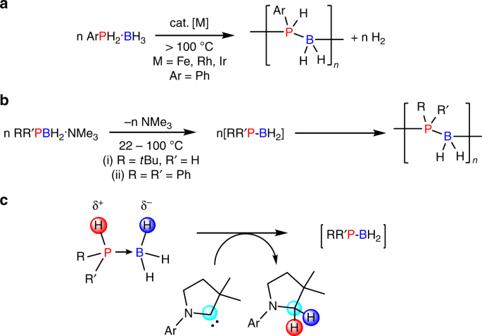Fig. 1 Synthesis of polyphosphinoboranes.a,bCurrent methods of synthesis andcproposed CAAC-mediated dehydrogenation The influence of temperature, solvent and concentration upon the molar mass of the poly(phenylphosphinoborane) obtained was systematically investigated with a view of optimising the polymerisation conditions (Table 1 ; Supplementary Table 1 ; and Supplementary Figs. 18 – 21 , 23 and 24 ). In each case, ESI-MS and gel permeation chromatography (GPC) analyses were carried out (Supplementary Figs. 11 – 17 , 22 and 23 ). ESI-MS clearly confirmed the presence of the [PhHPBH 2 ] monomeric repeat unit in each case and allowed us to detect the presence of either BH 3 or PPhH 2 end groups (Supplementary Fig. 22 ). However, due to only the low molar mass fraction being detected by the method, it is not possible to draw links between the reaction conditions and the degree of polymerisation using these data [47] . In contrast, GPC analysis permitted optimisation of the polymerisation conditions as this technique reveals the complete molar mass distribution (Table 1 and Supplementary Table 1 ). Increasing the temperature (run 1 vs. 3, and 5 vs. 6) reduced the reaction time, but has no significant effect on the molar mass of the polymer obtained. Using a non-polar solvent (toluene) rather than THF (runs 3 vs. 5) also had no significant effect on the polymer molar mass. It was found that at higher concentrations (run 2 vs. 3 vs. 4), a larger quantity of polymeric relative to oligomeric material was formed (Supplementary Fig. 17 ). This observation is consistent with head-to-tail polymerisation of transiently generated phenylphosphinoborane, [PhHPBH 2 ]. The reaction was also attempted under solvent-free, melt conditions at 110 °C (run 7), and, although high molar mass material was formed, the molar mass was no greater than that obtained using a concentrated solution at 60 °C. Due to concerns about the homogeneity of the reaction as a result of poor mixing, subsequent studies were performed in concentrated solutions rather than in the melt phase. Table 1 Influence of temperature, solvent and concentration on the formation of poly(phenylphosphinoborane), [PhHPBH 2 ] n , in a closed system Full size table Mechanistic studies A series of experimental and density functional theory (DFT) studies have been undertaken to probe the mechanism of the dehydrogenation of PhPH 2 ·BH 3 with CAAC Me . Several mechanisms for the generation of monomeric [PhHPBH 2 ] were considered and subsequently discounted, based on experimental and computational evidence (for a full discussion see ‘Proposed and subsequently discounted mechanisms for phosphine-borane dehydrogenation mediated by CAAC Me ’ in the Supplementary Information; Supplementary Figs. 32 and 33 ; and Supplementary Tables 3 and 5 ), before the final mechanism shown below was proposed and supported (Fig. 3 ). Attempts to trap the released monomer with either cyclohexene [48] or 1,3-cyclohexadiene [49] proved unsuccessful. Fig. 3 DFT study. Simplified schematic reaction profile calculated for the reaction of PhPH 2 ·BH 3 ( A ) with N -phenyl CAAC ( B ) at the PBE0/6-31 + G(d,p)/IEFPCM(THF) level of theory; Gibbs free energies for the second diastereomer are given in round brackets (for a comprehensive depiction of the reaction profile see Supplementary Fig. 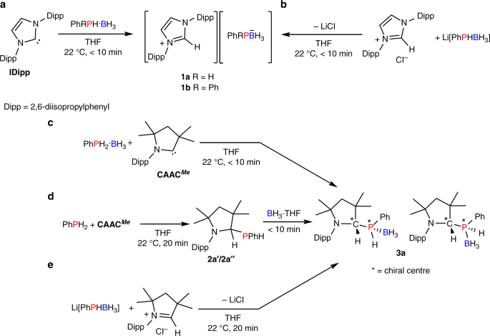Fig. 2 Reactivity of IDipp and CAACMewith phosphine-boranes.aSynthesis of1aand1bby deprotonation of the phosphine-borane using IDipp;bsynthesis of1aand1busing salt metathesis route;csynthesis of3athrough oxidative addition of PhPH2·BH3;dsynthesis of3athrough stepwise reaction of PhPH2, then BH3·THF; andesynthesis of3athrough salt metathesis route 31 ) Full size image Kinetic studies were conducted to assess the proposed mechanisms (Supplementary Table 2 and Supplementary Fig. 28 ). A plot of ln[ 3a ] vs. reaction time showed equivalent half-lives of 1.5 h (Supplementary Fig. 29 ) for several initial concentrations between 0.3 and 0.7 M at 50 °C, indicating a first-order process in 3a . Monitoring the reaction at several temperatures between 22 and 60 °C allowed the enthalpy and entropy of activation to be calculated as 21.5 kcal mol −1 and −9.5 cal K −1 mol −1 , respectively, consistent with a substantial energy barrier involving a relatively ordered transition state (Supplementary Fig. 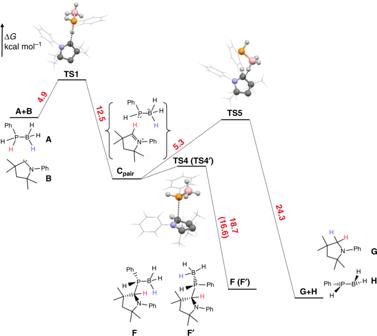Fig. 3 DFT study. Simplified schematic reaction profile calculated for the reaction of PhPH2·BH3(A) withN-phenyl CAAC (B) at the PBE0/6-31 + G(d,p)/IEFPCM(THF) level of theory; Gibbs free energies for the second diastereomer are given in round brackets (for a comprehensive depiction of the reaction profile see Supplementary Fig.31) 30 ). DFT calculations were carried out at the PBE0/6-31 + G(d,p)/IEFPCM(THF) level of theory [50] , [51] , [52] with an N -phenyl model system for the CAAC Me ( B ) to further elucidate the dehydrogenation mechanism (Fig. 3 ). An initial deprotonation of the P–H bond of PhPH 2 ·BH 3 ( A ) with B to give a [CAAC(H)] + and [PhPH(BH 3 )] − ion pair ( C pair ) was the most favoured first reaction step with a low Gibbs free energy of activation of 4.9 kcal mol −1 (see ‘DFT calculations’ in the Supplementary Information). Subsequent nucleophilic attack at the iminium carbon of the [CAAC(H)] + cation by the phosphorus centre of the [PhPH(BH 3 )] − anion leads via TS4 to the S P , S ( F ) diastereomer of the P–H activation product, or via TS4′ , to the other R P , S ( F′ ) diastereomer. The calculation of the activation barrier for this step was hampered by the inherently flat progression of the potential energy hypersurface between TS4 or TS4′ and C pair , which suggests, in agreement with the experimentally found rapid formation of 3a , that this step occurs with a very small activation barrier. F and F′ are kinetic products of the reaction. Significantly, this step is reversible via P–C dissociation, for which a maximum activation barrier of 18.7 kcal mol −1 was calculated from F to TS4 . This opens up a second reaction pathway from C pair leading to (CAAC)H 2 ( G ) and [PhHPBH 2 ] ( H ) via B–H hydride abstraction from the [PhPH(BH 3 )] − anion by the π-acidic (CAAC-H) + cation with a low activation barrier of 5.3 kcal mol −1 (via TS5 ). Thus, the formation of [PhHPBH 2 ] n from 3a can be rationalised by the formation of transient [CAAC(H)] + and [PhPH(BH 3 )] − ions via consecutive P–C bond scission and B–H hydride abstraction leading to (CAAC Me )H 2 and [PhHPBH 2 ], the latter undergoing head-to-tail polymerisation to thermodynamically favoured [PhHPBH 2 ] n (Supplementary Fig. 31 ). For a discussion of the proposed polymerisation mechanism, see ‘Supplementary discussion of the polymerisation mechanism from phosphinoborane monomers’ in the Supplementary Information. The fact that the reaction between PhPH 2 ·BH 3 and IDipp stops at the [IDipp(H)] + and [PhPH(BH 3 )] − ions (Fig. 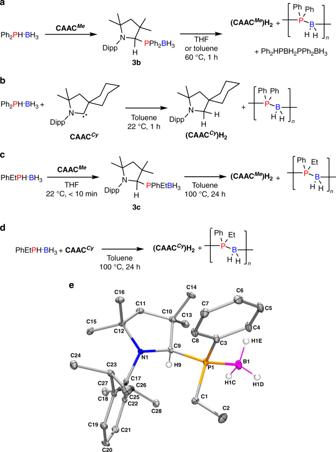Fig. 4 Reactions of Ph2PH·BH3andrac-Ph(Et)PH·BH3with CAACMeand CAACCy.aCAACMe-mediated dehydrocoupling of Ph2PH·BH3;bCAACCy-mediated dehydrocoupling of Ph2PH·BH3;cCAACMe-mediated dehydrocoupling ofrac-Ph(Et)PH·BH3;dCAACCy-mediated dehydrocoupling ofrac-Ph(Et)PH·BH3; andethermal ellipsoid plot of3c. H atoms other than those bound to C9 and B1 have been omitted for clarity. Ellipsoids are shown at the 30% probability level 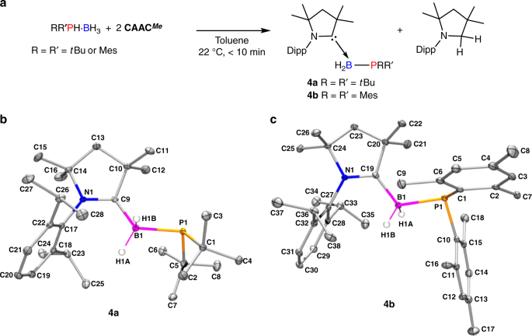Fig. 5 Synthesis and structure of cyclic (alkyl)(amino)carbene-phosphinoborane adducts4aand4b.aSynthesis of4aand4b;bthermal ellipsoid plot of4a; andcthermal ellipsoid plot of4b. For both4aand4bellipsoids are shown at the 30% probability level, and H atoms other than those at the B1 centre have been omitted for clarity 2a ) can be traced back to the greater π-acidity of the [CAAC(H)] + compared to the analogous [NHC(H)] + cation, as suggested by the high exergonicity of the isodesmic reaction [CAAC(H)] + + (NHC)H 2 → [NHC(H)] + + (CAAC)H 2 (Δ G 0 = −66.8 kcal mol −1 ; N -phenyl model systems) (Supplementary Table 4 ). According to the calculations, the dissociation of the P–H activation products F or F′ via the transition states TS4 or TS4′ requires the highest activation energy in the overall mechanism, which is in agreement with the first-order rate law found for 3a by the kinetic measurements. In addition, the calculated enthalpy of activation for this step (Δ H 0 = 20.2 ( TS4 ), 19.2 ( TS4′ ) kcal mol −1 ) is in good agreement with the substantial experimentally derived enthalpy of activation for the overall reaction (Δ H 0 = 21.5 kcal mol −1 ). The higher Gibbs free energy of activation required for the dissociation of the S P , S diastereomer F (Δ G 0 = 18.7 kcal mol −1 ) compared to the R P , S diastereomer F′ (Δ G 0 = 16.6 kcal mol −1 ) accounts for the experimentally observed faster conversion of one diastereomer during the reaction. Moreover, the observed enhanced reaction rates in THF (see Supplementary Table 2) can be rationalised by the better stabilisation of the [CAAC(H)] + and [PhPH(BH 3 )] − ions in THF than in toluene, which is further corroborated by the calculations (Supplementary Fig. 31 ). Substrate scope Given the success with PhPH 2 ·BH 3 , the scope of the CAAC Me -mediated dehydropolymerisation was extended with the aim of targeting hitherto inaccessible high molar mass P-disubstituted polyphosphinoboranes. CAAC Me (H)Ph 2 PBH 3 ( 3b ) was synthesised from Ph 2 PH·BH 3 and CAAC Me in THF (Fig. 4a and Supplementary Figs. 34 and 35 ). Formation of 3b was also detected immediately upon combining Li[Ph 2 PBH 3 ] and [CAAC Me H]Cl, and also through the stepwise addition of Ph 2 PH followed by BH 3 ·THF to a solution of CAAC Me . Fig. 4 Reactions of Ph 2 PH·BH 3 and rac -Ph(Et)PH·BH 3 with CAAC Me and CAAC Cy . a CAAC Me - mediated dehydrocoupling of Ph 2 PH·BH 3 ; b CAAC Cy - mediated dehydrocoupling of Ph 2 PH·BH 3 ; c CAAC Me -mediated dehydrocoupling of rac -Ph(Et)PH·BH 3 ; d CAAC Cy - mediated dehydrocoupling of rac -Ph(Et)PH·BH 3 ; and e thermal ellipsoid plot of 3c . H atoms other than those bound to C9 and B1 have been omitted for clarity. Ellipsoids are shown at the 30% probability level Full size image Heating a concentrated solution of 3b (2.5 M, 60 °C, 1 h, THF or toluene) effected complete conversion to (CAAC Me )H 2 , the linear dimer Ph 2 PHBH 2 PPh 2 BH 3 , cyclic oligomers [Ph 2 PBH 2 ] x ( x = 3, 4), and the polymer [Ph 2 PBH 2 ] n as observed by 1 H and 31 P NMR (Fig. 4a and Supplementary Fig. 40a ) [53] . Removal of (CAAC Me )H 2 and cyclic oligomers was achieved by precipitation into hexanes, but attempts to separate Ph 2 PHBH 2 PPh 2 BH 3 and [Ph 2 PBH 2 ] n proved unsuccessful (for details see ‘Dehydropolymerisation of Ph 2 PH·BH 3 ’ in the Supplementary Information). ESI-MS analysis of the product after precipitation nevertheless confirmed the presence of the repeat unit ∆( m/ z) = 198.08 (molecular weight of [Ph 2 PBH 2 ] = 198.08 g mol −1 , maximum value of n = 10) (Supplementary Fig. 36 ). However, GPC analysis showed only a very small amount of high molar mass material. Interestingly, when toluene, rather than THF, is used as the solvent, a much smaller quantity of linear dimer is formed (Supplementary Figs. 37 and 40b ). Under these conditions, GPC analysis on the precipitated material showed a majority of low molar mass material (M n = ca. 1,300; polydispersity index (PDI)  = 1.31) and a small amount (ca. 10%) of high molar mass material (M n = 54,300; PDI = 1.12) (Supplementary Fig. 38 ). With the aim of increasing the yield and amount of high molar mass material, we investigated the use of the more reactive CAAC Cy , exemplified by its ability to activate dihydrogen under mild conditions [37] . The initially formed P–H activation compound is consumed within 1 h at 22 °C (Fig. 4b ). However, GPC analysis again showed only a small amount (ca. 12%) of high molar mass material (M n = 59,600; PDI = 1.08) with the majority being low molar mass material (M n = ca. 1100; PDI = 1.28) (Supplementary Figs. 39 , 40c and 41 – 45 ). In an attempt to further extend the scope of the dehydropolymerisation to other P-disubstituted phosphine-boranes the reactivity of rac -Ph(Et)PH·BH 3 with CAAC Me and CAAC Cy was investigated. CAAC Me (H)PhEtPBH 3 ( 3c ) was formed through direct reaction of CAAC Me with rac -PhEtPH·BH 3 (Supplementary Figs. 46 – 50 ). Unlike with the mono- and di-phenyl derivatives, 3c is stable at 22 °C, which allowed the structure to be confirmed by X-ray diffraction (Fig. 4e and Supplementary Table 6 ). Upon heating isolated 3c to 100 °C, the targeted dehydropolymerisation occurred to give [PhEtPBH 2 ] n and (CAAC Me )H 2 (Fig. 4c and Supplementary Fig. 51 ). Pure [PhEtPBH 2 ] n was obtained in 23% yield as a fine white powder following precipitation. ESI-MS analysis of the precipitated sample confirmed the presence of the repeat unit of [PhEtPBH 2 ] n (∆( m/ z) = 150.08, molar mass of [PhEtPBH 2 ] = 150.08 g mol −1 ) and n = 33 (Supplementary Fig. 52 ); however, there was no convincing high molar mass material observed using GPC. In the analogous reaction using CAAC Cy , the yield was also low (19%); however, a GPC peak corresponding to high molar mass material (M n = 62,600, PDI = 1.19, n = ca. 400) was observed (Supplementary Figs. 53 – 58 ). Again this was only a small amount (ca. 18 %) compared to the low molar mass fraction (M n = ca. 1900; PDI = 1.47, n = ca. 13). Upon closer analysis of the ESI-MS spectra for each synthesis of [Ph 2 PBH 2 ] n and [PhEtBH 2 ] n , the end group of the major distribution was detected as being either CAAC Me or CAAC Cy (Supplementary Figs. 36 , 37 , 44 , 52 and 56 ). These results suggest that trace amounts of CAACs may react with the polymer chain at some point during the polymerisation (for further discussion see ‘Supplementary discussion of the polymerisation mechanism from phosphinoborane monomers’ in the Supplementary Information). When the reactivity of CAAC Me with bulkier P-disubstituted phosphine-borane substrates (R = R′ = t Bu or R = R′ = Mes) was explored, an enlightening divergence in reactivity was noted. For full conversion of these substrates, two equivalents of CAAC Me are required. In situ 1 H NMR reveals that an equimolar mixture of (CAAC Me )H 2 and the new species 4a / 4b are formed (Fig. 5a and Supplementary Figs. 59 – 68 ). Fig. 5 Synthesis and structure of cyclic (alkyl)(amino)carbene-phosphinoborane adducts 4a and 4b . a Synthesis of 4a and 4b ; b thermal ellipsoid plot of 4a ; and c thermal ellipsoid plot of 4b . For both 4a and 4b ellipsoids are shown at the 30% probability level, and H atoms other than those at the B1 centre have been omitted for clarity Full size image The structures of 4a and 4b were confirmed by X-ray crystallography revealing that in both compounds the CAAC Me C-donor was bound to the boron of the phosphinoborane moiety (Fig. 5b, c and Supplementary Table 7 ). Interestingly, species 4a and 4b are analogous to the previously mentioned NHC–phosphinoborane adducts that have been recently reported [45] . The reactivity with the bulky, P-disubstituted phosphine-boranes contrasts with that observed with PhPH 2 ·BH 3 , Ph 2 PH·BH 3 and PhEtPH·BH 3 as an initial P–H oxidative-addition product analogous to compounds 3a–c is not observed. The monomeric phosphinoborane generated upon dehydrogenation does not undergo head-to-tail polymerisation, instead it is trapped by a second equivalent of carbene. The absence of an observable P–H activation compound can be explained by the greater steric bulk around the phosphorus centre. The trapping, however, provides further evidence for the release of monomeric phosphinoboranes in the proposed polymerisation mechanism. It is noteworthy that when Ph 2 PH·BH 3 is reacted with two equivalents of CAAC Me clean conversion to the species analogous to 4a and 4b is not observed; however, peaks for the short-chain oligomers CAAC(BH 2 PPh 2 ) x ( x = 1–4) have been identified using ESI-MS (Supplementary Fig. 69 ). In summary, we have shown that cyclic alkyl(amino)carbenes can be used as stoichiometric reagents to effect P–H/B–H dehydrogenative coupling of primary and secondary phosphine-boranes. These results illustrate the complementarity between organic and transition metal ambiphiles in the context of the main-group redox transformations, and hint at a potentially broad utility for CAACs in accessing new inorganic polymers and materials. The carbene centre in CAAC Me inserts into the P–H bond of phosphine-boranes, RR′PH·BH 3 (R = Ph; R′ = H, Ph, or Et), to give derivatives of CAAC Me (H)PRR′BH 3 ( 3a–c ) which undergo thermolysis to give the hydrogenated carbene (CAAC Me )H 2 and polymers [RR′PBH 2 ] n . Most remarkable is that in the case of Ph 2 PH·BH 3 with CAAC Cy the dehydropolymerisation proceeds within 1 h at 22 °C. In contrast, with respect to the reactivity of sterically encumbered P-disubstituted phosphine-boranes (R = R′ = t Bu or Mes) with CAAC Me , it is noteworthy that polymers are not generated post H 2 transfer. Instead, the transient phosphinoboranes were trapped by a second equivalent of carbene to yield CAAC Me –phosphinoborane adducts, 4a and 4b . The novel dehydropolymerisation using CAACs has been used to prepare samples of P-disubstituted polyphosphinoboranes, [Ph 2 PBH 2 ] n and [PhEtPBH 2 ] n , which cannot be accessed via previous transition metal-catalysed or stoichiometric routes, and contain high molar mass fractions. The development of catalytic rather than stoichiometric reactions involving main-group species is a rapidly developing field [54] , [55] . The reactions of phosphine-boranes with species that undergo E–H bond activation, for example, stannylenes [56] and frustrated Lewis pairs that reversibly bind H 2 [57] , [58] , are under current investigation. Future studies will target the generation of a well-defined propagating site, which should allow access to predominantly linear polymers, molar mass control and potentially block copolymers. A more atom-economic catalytic synthesis would also allow a more facile scale-up and thereby the properties of the new materials to be investigated in detail. Detailed procedure for polymerisation of PhPH 2 · BH 3 using CAAC Me (run 4) PhPH 2 · BH 3 (156 mg, 1.26 mmol) and CAAC Me (360 mg, 1.26 mmol) were dissolved in THF (1 mL) in a J. Young Schlenk tube, sealed and the reaction mixture was stirred at 60 °C for 3 h. The reaction mixture was added dropwise into 20 mL of rapidly stirred cold hexanes at −40 °C, yielding a precipitate, and the supernatant was decanted. The precipitation was repeated twice more prior to drying in vacuo to leave a white powder of the [PhHPBH 2 ] n polymer product. Yield (precipitated material) = 42 mg (27%). GPC (2 mg mL −1 ): M n = 83,800 Da; PDI = 1.17. Full experimental details for all polymerisations can be found in the Supplementary Methods.